Phytochrome-interacting transcription factors PIF4 and PIF5 induce leaf senescence inArabidopsis Plants initiate senescence to shed photosynthetically inefficient leaves. Light deprivation induces leaf senescence, which involves massive transcriptional reprogramming to dismantle cellular components and remobilize nutrients. In darkness, intermittent pulses of red light can inhibit senescence, likely via phytochromes. However, the precise molecular mechanisms transducing the signals from light perception to the inhibition of senescence remain elusive. Here, we show that in Arabidopsis , dark-induced senescence requires phytochrome-interacting transcription factors PIF4 and PIF5 (PIF4/PIF5). ELF3 and phytochrome B inhibit senescence by repressing PIF4/PIF5 at the transcriptional and post-translational levels, respectively. PIF4/PIF5 act in the signalling pathways of two senescence-promoting hormones, ethylene and abscisic acid, by directly activating expression of EIN3 , ABI5 and EEL . In turn, PIF4, PIF5, EIN3, ABI5 and EEL directly activate the expression of the major senescence-promoting NAC transcription factor ORESARA1 , thus forming multiple, coherent feed-forward loops. Our results reveal how classical light signalling connects to senescence in Arabidopsis . Leaf senescence, the final stage of leaf development, actively destabilizes intracellular organelles, including decomposition of macromolecules, to relocate nutrients into developing tissues or storage organs. Senescence occurs autonomously in an age-dependent manner, controlled by an innate genetic programme. However, unfavorable environmental stresses, such as darkness, drought, high temperature, high salinity and pathogen attacks, can also trigger senescence during leaf development [1] . For example, light deprivation induces senescence in lower leaves that are shaded by upper leaves [2] . Molecular genetic studies using Arabidopsis thaliana have identified many senescence-associated genes (SAGs), including genes involved in hormone signalling, transcriptional regulation and chlorophyll (Chl) catabolism [1] , [3] . The developmental and environmental signals of senescence commonly activate senescence-associated transcriptional factors (senTFs), which modulate the expression of SAGs [4] . To date, transcriptome analyses and molecular genetic studies, in Arabidopsis and other plants, have identified many senTFs [3] , [5] . In particular, the senTFs include a few plant-specific NAC genes, such as ORESARA1 ( ORE1 , also known as NAC092 ) [5] , indicating that the senescence-induced NAC transcription factors have important roles in modulating senescence. ORE1 promotes senescence by regulating the expression of hundreds of SAGs that function in the breakdown of nucleic acids and proteins, and the transport of sugar [6] , [7] . Treatment with ethylene or abscisic acid (ABA) upregulates ORE1 expression [8] , suggesting a close relationship between hormone signalling and ORE1 . Among the senescence-induced NACs, NAC-LIKE, ACTIVATED BY AP3/PI ( NAP/NAC029 ) and NAC016 also promote senescence, as demonstrated by the delayed senescence phenotype of nap and nac016 mutants [9] , [10] . In contrast, JUNGBRUNNEN 1 ( JUB1/NAC042 ) and VND-INTERACTING 2 ( VNI2/NAC083 ) inhibit leaf senescence [11] , [12] . Thus, these observations show that the senescence-promoting and senescence-inhibiting NACs finely tune the expression of SAGs in response to developmental and environmental cues. Plant hormones coordinate senescence in connection with senTFs, and ensure that senescence proceeds in an orderly fashion at the organismal level. Among plant hormones, ethylene promotes senescence, as demonstrated by accelerated senescence in ethylene-treated plants [13] and delayed senescence in mutants impaired in ethylene signalling, including mutants in the ethylene signalling component ETHYLENE INSENSITIVE 2 ( EIN2 ), the transcription factor EIN3 and the ethylene receptor ETHYLENE INSENSITIVE 1 ( ETR1 ) (refs 14 , 15 , 16 ). ABA also induces senescence rapidly [17] . Mutants of RECEPTOR-LIKE PROTEIN KINASE 1 ( RPK1 ) and SENESCENCE-ASSOCIATED GENE 113 ( SAG113 ), which are insensitive to ABA, display delayed senescence phenotypes [18] , [19] . Senescence is rapidly induced by treatment with salicylic or jasmonic acids [20] , [21] , but is extremely delayed by cytokinin treatment [22] . The exact molecular mechanisms of how these hormone signals coordinate the ageing or stress signals for leaf senescence are not fully understood. Plant growth and development requires light [23] , and plants require photoreceptors to adapt to ambient light conditions throughout development. Red light has long been considered to be a key negative signal for plant senescence, because pulses of red light substantially delay dark-induced senescence (DIS) in a few plant species, supposedly via phytochromes [24] and a low ratio of red/far-red light causes senescence in tobacco leaves [25] . Red light activates and far-red light inactivates phytochromes; darkness also causes slow inactivation of phytochromes [23] . Photoactivated phytochromes move from the cytosol to the nucleus, where they interact with and inactivate the negative regulators of light signalling, resulting in massive transcriptome changes [23] . In Arabidopsis , phyA and phyB regulate a wide range of light responses such as seed germination, seedling photomorphogenesis, hypocotyl gravitropism, shade avoidance and flowering time [23] . Phytochromes inactivate phytochrome-interacting bHLH transcription factors (PIFs), which inhibit light responses in the dark [26] . At the molecular level, active phytochromes directly interact with PIFs to induce their detachment from DNA [27] , and promote their degradation by the 26S proteasome [28] , [29] . PIFs are also regulated at the transcriptional level; the EARLY FLOWERING 3 (ELF3)-ELF4- LUX ARRHYTHMO (LUX) complex directly associates with the promoters of PIF4 and PIF5 ( PIF4/PIF5 ) and suppresses their expression in the regulation of circadian responses [30] . Although the regulatory function of the phytochrome-PIF signalling module has been intensively investigated in the light-responsive development of Arabidopsis seedlings, it is unknown if this signalling module has a role in plant senescence. Here, we show the molecular mechanism of how the phytochrome-PIF signalling module activates leaf senescence in Arabidopsis . We found that among the four PIFs, PIF4/PIF5 function as the essential, central transcriptional activators of DIS and that ELF3 and red light-activated phyB repress the senescence-promoting activity of PIF4/PIF5 at the transcriptional and post-translational levels, respectively. The two PIFs activate the expression of ORE1 by forming multiple coherent feed-forward loops, together with two distinct classes of transcription factors, EIN3 in ethylene signalling and Group A bZIPs (ABA INSENSITIVE 5 (ABI5) and ENHANCED EM LEVEL (EEL)) in ABA signalling. The Pfr form of phyB inhibits leaf senescence Phytochromes are red/far-red photoreceptors that can be interconverted to active Pfr and inactive Pr forms by red and far-red light irradiation, respectively [31] . To examine the effect of phytochrome-mediated light signalling on leaf senescence, 7-day-old Arabidopsis wild-type (WT) seedlings were incubated for 10-day in darkness (control), and in darkness with intermittent pulses of red light (phyB on ) or with pulses of red light followed by far-red light (phyB off ) ( Fig. 1a , left panel). WT cotyledons turned yellow during dark incubation, a typical symptom of senescence in plants. When the light pulses were given, we found that the cotyledons stayed green in phyB on conditions but turned yellow in phyB off conditions ( Fig. 1a , right panel), indicating that the Pfr form of phyB inhibits senescence. To investigate the role of phyB in senescence, we examined the phenotypes of 7-day-old seedlings of phyB mutants and PHYB -overexpressing ( PHYB -OX) plants after 8 days of dark incubation (DDI). phyB mutants senesced faster and PHYB -OX plants senesced slower than WT ( Fig. 1b,e,f ). Similar to the seedling phenotypes, when attached or detached leaves of 3-week-old plants were incubated in darkness or individual leaves were covered with aluminium foil under long day conditions, phyB mutants senesced faster and PHYB -OX plants senesced slower than WT ( Fig. 1c,d ; Supplementary Fig. 1a and Supplementary Methods ). Consistent with their visible phenotypes, phyB mutants had lower Chl levels, higher ion leakage rates, higher expression of two senescence marker genes ( SENESCENCE 4 ( SEN4 ) and SAG12 ), and lower expression of a photosynthetic gene ( LIGHT HARVESTING CHLOROPHYLL A/B BINDING PROTEIN 1 ( Lhcb1 )) than WT seedlings or individually covered leaves of adult plants during dark incubation, while PHYB -OX had the opposite phenotypes, with the exception of ion leakage rate ( Fig. 1e–g , Supplementary Fig. 1b–d ). It appears that PHYB overexpression is not sufficient to retard the breakdown of membrane integrity of seedlings during DIS. In contrast, phyA mutants and PHYA -OX plants senesced at the same rate as WT ( Supplementary Fig. 2 ). The results indicate that phyB is the major photoreceptor signalling to suppress senescence in Arabidopsis . 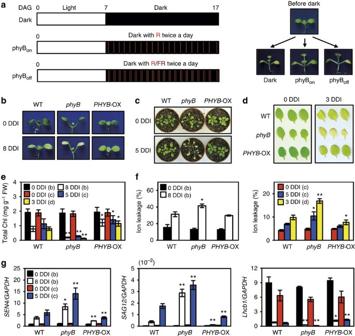Figure 1: PhyB suppresses senescence. (a) Suppression of senescence by treatment with intermittent red light pulses during dark incubation. Light-grown 7-day-old WT (Col-0 ecotype) seedlings were transferred to darkness for 10 days without any light (continuous darkness), with intermittent red light pulses (phyBon) or with red light pulses immediately followed by far-red light pulses (phyBoff). R and FR indicate red light and far-red light pulses, respectively. (b–f) Suppression of senescence by phyB as judged by changes in leaf colour. Light-grown 7-day-old WT (Col-0),phyB(phyB-9) andPHYB-OX seedlings (b), and attached (c) or detached leaves (d) of 3-week-old WT,phyBandPHYB-OX plants were transferred to darkness for the indicated number of days. Total Chl levels (e) and ion leakage rates (f) in (b–d) were determined before and after dark treatment. (g) Expression levels ofSEN4,SAG12andLhcb1of WT,phyBandPHYB-OX in 7-day-old seedlings or 3-week-old plants during dark incubation. For quantitative real-time PCR, the relative expression levels were determined by normalizing to the transcript levels ofGAPDH.PHYB-OX indicates the plants (Col) overexpressingPHYBunder the control of 35S promoter. Mutant information is listed inSupplementary Table 3. Data are means±s.d. of more than four independent biological replicates. *P<0.05, **P<0.01 (Student’st-test). DAG, day(s) after germination. Figure 1: PhyB suppresses senescence. ( a ) Suppression of senescence by treatment with intermittent red light pulses during dark incubation. Light-grown 7-day-old WT (Col-0 ecotype) seedlings were transferred to darkness for 10 days without any light (continuous darkness), with intermittent red light pulses (phyB on ) or with red light pulses immediately followed by far-red light pulses (phyB off ). R and FR indicate red light and far-red light pulses, respectively. ( b – f ) Suppression of senescence by phyB as judged by changes in leaf colour. Light-grown 7-day-old WT (Col-0), phyB ( phyB-9 ) and PHYB -OX seedlings ( b ), and attached ( c ) or detached leaves ( d ) of 3-week-old WT, phyB and PHYB -OX plants were transferred to darkness for the indicated number of days. Total Chl levels ( e ) and ion leakage rates ( f ) in ( b – d ) were determined before and after dark treatment. ( g ) Expression levels of SEN4 , SAG12 and Lhcb1 of WT, phyB and PHYB -OX in 7-day-old seedlings or 3-week-old plants during dark incubation. For quantitative real-time PCR, the relative expression levels were determined by normalizing to the transcript levels of GAPDH . PHYB -OX indicates the plants (Col) overexpressing PHYB under the control of 35S promoter. Mutant information is listed in Supplementary Table 3 . 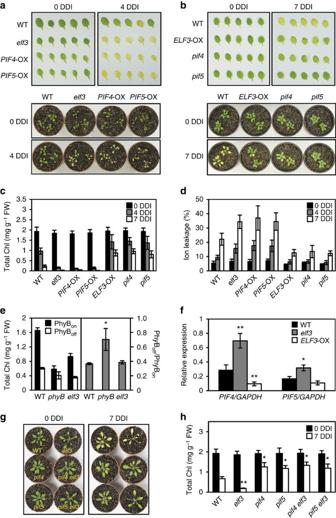Figure 3: ELF3 inhibits senescence. (a–d) Inhibition of senescence by ELF3 in darkness. Three-week-old detached leaves (upper) or whole plants (lower) grown in long days were transferred to complete darkness and photographed at 4 DDI (a) or at 7 DDI (b). Total Chl levels (c) and ion leakage rates (d) were measured at indicated DDIs.elf3iself3-8(Supplementary Table 3).PIF4-OX,PIF5-OX andELF3-OX indicate the plants overexpressingPIF4,PIF5andELF3under the control of 35S promoter, respectively. (e) Independent regulation of senescence by ELF3 and phyB. The 7-day-old seedlings grown in continuous light conditions were transferred to darkness for 16 days with intermittent red (PhyBon) or red/far-red light pulses (PhyBoff) as shown inFig. 1a. phyBoff/phyBonindicates that total Chl levels of WT,phyBandelf3mutants in PhyBoffconditions are normalized to those in PhyBonconditions. (f) Repression ofPIF4/PIF5transcription by ELF3. The 7-day-old WT (black bars),elf3mutants (red bars) andELF3-OX plants (blue bars) were transferred to darkness for 2 days.PIF4/PIF5expression was normalized toGAPDHexpression. (g,h)PIF4/PIF5are epistatic toELF3. Three-week-old plants grown in long days were transferred to darkness for 7 days (g) and total Chl levels were measured (h). DDI indicates day(s) of dark incubation. Data are means±s.d. of at least four biological replicates. *P<0.05, **P<0.01 (Student’st-test). Data are means±s.d. of more than four independent biological replicates. * P <0.05, ** P <0.01 (Student’s t -test). DAG, day(s) after germination. Full size image Mutations in PIF4 and PIF5 delay leaf senescence We next investigated which phyB signalling components regulate DIS in Arabidopsis leaves. Previous work showed that pif quadruple ( pifQ ) mutants ( pif1 pif3 pif4 pif5 ) show a constitutive photomorphogenic phenotype when grown in darkness, and phyB promotes light responses by repressing the activity of PIFs [32] , [33] . We found that pifQ mutants maintained green cotyledons at 10 DDI, while WT cotyledons turned completely yellow ( Fig. 2a ), indicating that PIFs promote senescence in light-deprived conditions. To determine which PIFs promote senescence, we examined the seedling phenotypes of four pif single mutants during dark incubation. The pif1 and pif3 mutants turned yellow at the same rate as WT, but pif4 and pif5 mutants, similar to pifQ mutants, senesced slower than WT ( Fig. 2b ). We also observed a similar delayed senescence pattern in the attached, detached or individually covered leaves of pif4 , pif5 and pifQ mutants ( Fig. 2c,d ; Supplementary Fig. 3a ). Consistent with their visible phenotypes, the mutants had higher Chl levels, lower ion leakage rates, lower expression of SEN4 and higher expression of Lhcb1 than WT ( Supplementary Figs 3b,c, 4 and 5 ). In addition, pifQ mutants maintained better-preserved chloroplast structure and pif4 and pif5 mutants retained higher levels of photosystem proteins ( Supplementary Fig. 6 and Supplementary Methods ). Moreover, PIF4/PIF5 also promote age-dependent leaf senescence, as pif4 and pif5 mutant leaves senesced slower than WT leaves under long days ( Supplementary Fig. 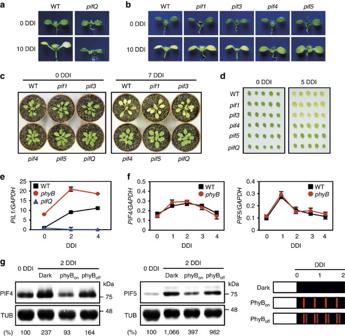7 ), suggesting that PIF4/PIF5 are the essential transcription factors that promote leaf senescence under not only dark-induced, but also under natural senescence conditions. Figure 2: PIF4 and PIF5 (PIF4/PIF5) promote senescence. (a–d) Delayed senescence ofpif4andpif5mutants in darkness. WT andpifQindicate wild-type (Col-0) andpif1 pif3 pif4 pif5quadruple mutants, respectively. For the assay, 7-day-old seedlings were grown in continuous light (a,b), and attached (c) or detached (4th or 5th) leaves (d) of 3-week-old plants grown under long days were incubated in darkness and photographed. Mutant information is listed inSupplementary Table 3. (e)PIL1expression in WT (black line),phyBmutants (phyB-9; red line), andpifQmutants (blue line) during dark incubation. Means±s.d. were calculated from at least four independent replicates. (f)PIF4/PIF5expression in WT (black lines) andphyBmutants (red lines) during dark incubation. (e,f) By reverse transcription and quantitative real-time PCR, relative transcript levels ofPIL1(e) andPIF4/PIF5(f) were normalized to those ofGAPDH(a control). (g) Stabilization of PIF4/PIF5 proteins in phyBoffconditions. The 35S-driven PIF4/PIF5-Myc and tubulin (TUB; a control) were detected by anti-Myc and anti-tubulin antibodies, respectively. PIF4/PIF5 levels were normalized to TUB protein levels. Figure 2: PIF4 and PIF5 (PIF4/PIF5) promote senescence. ( a – d ) Delayed senescence of pif4 and pif5 mutants in darkness. WT and pifQ indicate wild-type (Col-0) and pif1 pif3 pif4 pif5 quadruple mutants, respectively. For the assay, 7-day-old seedlings were grown in continuous light ( a , b ), and attached ( c ) or detached (4th or 5th) leaves ( d ) of 3-week-old plants grown under long days were incubated in darkness and photographed. Mutant information is listed in Supplementary Table 3 . ( e ) PIL1 expression in WT (black line), phyB mutants ( phyB-9 ; red line), and pifQ mutants (blue line) during dark incubation. Means±s.d. were calculated from at least four independent replicates. ( f ) PIF4/PIF5 expression in WT (black lines) and phyB mutants (red lines) during dark incubation. ( e , f ) By reverse transcription and quantitative real-time PCR, relative transcript levels of PIL1 ( e ) and PIF4/PIF5 ( f ) were normalized to those of GAPDH (a control). ( g ) Stabilization of PIF4/PIF5 proteins in phyB off conditions. The 35S-driven PIF4/PIF5-Myc and tubulin (TUB; a control) were detected by anti-Myc and anti-tubulin antibodies, respectively. PIF4/PIF5 levels were normalized to TUB protein levels. Full size image To gauge if PIF4/PIF5 transcription factors become active during dark incubation, we examined the expression of the PIF target gene PHYTOCHROME-INTERACTING FACTOR 3-LIKE 1 ( PIL1 ) during dark incubation, as PIFs directly regulate PIL1 expression [34] . PIL1 mRNA levels increased and plateaued at 2 DDI in WT ( Fig. 2e ). However, PIL1 mRNA levels did not rise in pifQ mutants; in contrast, phyB mutants showed much higher PIL1 mRNA levels than WT. The altered expression of PIL1 in pifQ and phyB mutants provides indirect evidence that phyB negatively regulates the activity of PIF4/PIF5 in the light; the increased activity of PIF4/PIF5 in the prolonged darkness could be caused by the increase of PIF4/PIF5 transcription, PIF4/PIF5 protein stability or both. To investigate this, we first examined the expression levels of PIF4/PIF5 during dark incubation and found that their expression in phyB mutants was almost the same as in WT ( Fig. 2f ). This suggests that phyB does not regulate PIF4/PIF5 at the transcriptional level, but may possibly act at the post-translational level. Indeed, we found that in PIF4 -OX and PIF5 -OX plants, the levels of PIF4/PIF5 proteins increased in darkness ( Fig. 2g ). Intermittent pulses of red light (PhyB on ) inhibited the increase of PIF4/PIF5 proteins, but pulses of red light followed by far-red light (PhyB off ) did not, indicating that the PIF4/PIF5 proteins are stabilized when phyB converts to the inactive Pr form. ELF3 inhibits leaf senescence by repressing PIF4/PIF5 A previous study showed that an ELF3–ELF4–LUX complex represses the expression of PIF4/PIF5 in the evening phase [30] . Thus, we examined if ELF3 inhibits leaf senescence by repressing PIF4/PIF5 transcription during dark incubation. We found that elf3 mutants, similar to PIF4 -OX and PIF5 -OX plants, senesced much faster than WT in both detached and attached leaves of adult plants ( Fig. 3a ; Supplementary Fig. 8a ), while ELF3 -OX plants, similar to pif4 and pif5 mutants, exhibited delayed senescence ( Fig. 3b ), as shown by Chl levels ( Fig. 3c ), ion leakage rates ( Fig. 3d ), the expression levels of SEN4 and Lhcb1 ( Supplementary Fig. 5 ) and chloroplast structure and photosystem protein levels ( Supplementary Fig. 6 ). ELF3 functions as one of the critical factors in light input into the circadian clock and in the regulation of flowering time [35] , [36] ; therefore, we further examined whether senescence is also affected by mutations of other regulators of the circadian clock, flowering time and photomorphogenesis, such as CIRCADIAN-CLOCK ASSOCIATED 1 ( CCA1 ), LATE ELONGATED HYPOCOTYL ( LHY ), ELF4 , LUX , FLAVIN-BINDING, KELCH REPEAT, F-BOX 1 ( FKF1 ), CRYPTOCHROME 2 ( CRY2) , GIGANTEA ( GI ), CONSTANS ( CO ), CONSTITUTIVE PHOTOMORPHOGENIC 1 ( COP1 ) and DE-ETIOLATED 1 ( DET1 ) (refs 36 , 37 ). We found that none of the mutants for these regulators showed altered senescence phenotypes during dark incubation ( Supplementary Fig. 8b ). Although CRY1 was suggested to regulate PIF4/PIF5 for shade avoidance responses [38] , we found that detached leaves of cry1 , cry2 and cry1 cry2 double mutants did not show an early or delayed senescence phenotype during dark incubation ( Supplementary Fig. 8c ). These results indicate that among the components we tested, ELF3 functions as a unique negative regulator of senescence induction. Figure 3: ELF3 inhibits senescence. ( a – d ) Inhibition of senescence by ELF3 in darkness. Three-week-old detached leaves (upper) or whole plants (lower) grown in long days were transferred to complete darkness and photographed at 4 DDI ( a ) or at 7 DDI ( b ). Total Chl levels ( c ) and ion leakage rates ( d ) were measured at indicated DDIs. elf3 is elf3-8 ( Supplementary Table 3 ). PIF4 -OX, PIF5 -OX and ELF3 -OX indicate the plants overexpressing PIF4 , PIF5 and ELF3 under the control of 35S promoter, respectively. ( e ) Independent regulation of senescence by ELF3 and phyB. The 7-day-old seedlings grown in continuous light conditions were transferred to darkness for 16 days with intermittent red (PhyB on ) or red/far-red light pulses (PhyB off ) as shown in Fig. 1a . phyB off /phyB on indicates that total Chl levels of WT, phyB and elf3 mutants in PhyB off conditions are normalized to those in PhyB on conditions. ( f ) Repression of PIF4/PIF5 transcription by ELF3. The 7-day-old WT (black bars), elf3 mutants (red bars) and ELF3 -OX plants (blue bars) were transferred to darkness for 2 days. PIF4/PIF5 expression was normalized to GAPDH expression. ( g , h ) PIF4/PIF5 are epistatic to ELF3 . Three-week-old plants grown in long days were transferred to darkness for 7 days ( g ) and total Chl levels were measured ( h ). DDI indicates day(s) of dark incubation. Data are means±s.d. of at least four biological replicates. * P <0.05, ** P <0.01 (Student’s t -test). Full size image ELF3 acts as a phyB signalling component in seedling development [35] ; we thus tested whether ELF3 inhibits senescence through red light-activated phyB signalling. Although both phyB and elf3 mutants senesced faster than WT, elf3 mutants still responded to red light pulses comparable to WT, whereas phyB mutants did not ( Fig. 3e ), indicating that ELF3 suppresses DIS independent of phyB. Since the expression of PIF4/PIF5 increased during dark incubation independent of phyB activity ( Fig. 2f ), we measured the mRNA levels of PIF4/PIF5 in elf3 mutants and ELF3 -OX plants at 2 DDI ( Fig. 3f ). We found that the PIF4 expression was higher in elf3 mutants than in WT, and lower in ELF3 -OX plants. PIF5 expression also increased more in elf3 mutants. Furthermore, the pif4 elf3 and pif5 elf3 double mutants senesced much later than WT, but similar to pif4 and pif5 single mutants at 7 DDI ( Fig. 3g,h ), demonstrating that pif4 and pif5 are epistatic to elf3 . Consistent with this, ELF3 -OX PIF4 -OX plants senesced faster than WT, but similar to PIF4 -OX plants ( Supplementary Fig. 9 ). These results indicate that ELF3 represses PIF4/PIF5 transcription independent of phyB, while the Pfr form of phyB destabilizes PIF4/PIF5 proteins. PIF4/PIF5 promote ethylene and ABA signalling To investigate how PIF4/PIF5 promote DIS at the molecular level, we performed microarray analysis and identified 677 differentially expressed genes (DEGs) between WT and pifQ mutants at 2 DDI (WT/ pifQ , twofold, false discovery rate (FDR)<0.05; Fig. 4a , left circle). We compared the DEGs of WT/ pifQ with those of senescing WT at 2 DDI (DIS (2 days/0 days)) ( Fig. 2a , right circle) from previously reported microarray data [39] . We found that the two sets share 132 DEGs ( P <10 −72 , hypergeometric test), showing a high correlation coefficient ( R =0.85; Supplementary Fig. 10a ). The common DEGs have enriched functional categories of ageing, leaf senescence, photosynthesis, Chl metabolism and light response ( Supplementary Fig. 10b ). Moreover, although the changes were less than twofold, Gene Set Enrichment Analysis (GSEA, see Methods) showed that the non-shared DEGs of senescing WT also significantly correlated with the changes in pifQ mutants ( Supplementary Fig. 10c ). The results indicate that PIF4/PIF5 function as the major regulators of SAG expression in senescing leaves during dark incubation. 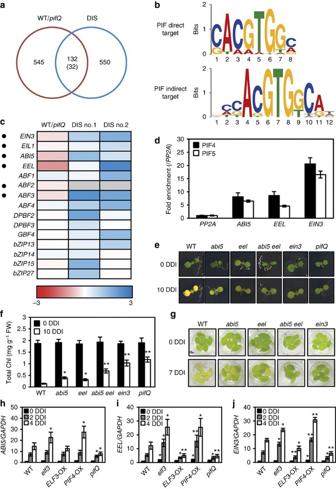Figure 4: PIF4/PIF5 directly induce bZIPs andEIN3. (a) Significant overlap between DEGs (twofold, FDR<0.05) of PIF-induced genes (WT/pifQ, this study) and DIS genes (previous microarray data39). Light-grown 7-day-old WT andpifQseedlings were transferred to darkness for 2 days (WT versuspifQ), and 4-week-old adult WT plants were transferred to darkness for 0 and 2 days (2 DDI versus 0 DDI). The number in parentheses indicates the PIF4/PIF5-direct target genes retrieved from the previous ChIP-seq database34,40. (b) Enrichment of the G-box motifs in the PIF-direct target promoters and the ABRE-like element in the PIF-indirect target promoters, identified by the MEME software using 500 bp promoter sequences. (c) Heat map showing the expression ofEIN3,EIL1and group A bZIPs in the microarray analysis from this study (WT/pifQ) and two independent sets of DIS microarray data from previous studies39,69. Black circles indicate the PIF4/PIF5-direct target genes according to previous ChIP-seq analyses34,40. The scale bar (bottom) indicates fold changes as log2values. TheABF2probe is absent in the DIS microarray (Affymetrix). (d) Direct binding of PIF4/PIF5 to the promoters ofABI5,EELandEIN3by ChIP assays. Values were normalized to the values forPP2Aas a non-binding control. Data are means±s.d. of two biological replicates. (e–g) Delayed senescence ofabi5,eel,abi5 eel,ein3andpifQmutants. Light-grown 7-day-old seedlings were transferred to darkness for 10 days (e). Total Chl levels were measured at 10 DDI (f). Data are means±s.d. of at least four biological replicates. Detached leaves of 3-week-old plants were transferred to darkness and photographed at 7 DDI (g). (h–j) Regulation ofABI5, EELandEIN3expression by ELF3 and PIF4/5. The mRNA levels were determined by quantitative real-time PCR using light-grown 7-day-old seedlings transferred to darkness for 0, 2 and 4 DDI.GAPDHwas used as a control. DDI indicates day(s) of dark incubation. Data are means±s.d. of four biological replicates. *P<0.05, **P<0.01 (Student’st-test). Figure 4: PIF4/PIF5 directly induce bZIPs and EIN3. ( a ) Significant overlap between DEGs (twofold, FDR<0.05) of PIF-induced genes (WT/ pifQ , this study) and DIS genes (previous microarray data [39] ). Light-grown 7-day-old WT and pifQ seedlings were transferred to darkness for 2 days (WT versus pifQ ), and 4-week-old adult WT plants were transferred to darkness for 0 and 2 days (2 DDI versus 0 DDI). The number in parentheses indicates the PIF4/PIF5-direct target genes retrieved from the previous ChIP-seq database [34] , [40] . ( b ) Enrichment of the G-box motifs in the PIF-direct target promoters and the ABRE-like element in the PIF-indirect target promoters, identified by the MEME software using 500 bp promoter sequences. ( c ) Heat map showing the expression of EIN3 , EIL1 and group A bZIPs in the microarray analysis from this study (WT/ pifQ ) and two independent sets of DIS microarray data from previous studies [39] , [69] . Black circles indicate the PIF4/PIF5-direct target genes according to previous ChIP-seq analyses [34] , [40] . The scale bar (bottom) indicates fold changes as log 2 values. The ABF2 probe is absent in the DIS microarray (Affymetrix). ( d ) Direct binding of PIF4/PIF5 to the promoters of ABI5 , EEL and EIN3 by ChIP assays. Values were normalized to the values for PP2A as a non-binding control. Data are means±s.d. of two biological replicates. ( e – g ) Delayed senescence of abi5 , eel , abi5 eel , ein3 and pifQ mutants. Light-grown 7-day-old seedlings were transferred to darkness for 10 days ( e ). Total Chl levels were measured at 10 DDI ( f ). Data are means±s.d. of at least four biological replicates. Detached leaves of 3-week-old plants were transferred to darkness and photographed at 7 DDI ( g ). ( h – j ) Regulation of ABI5, EEL and EIN3 expression by ELF3 and PIF4/5. The mRNA levels were determined by quantitative real-time PCR using light-grown 7-day-old seedlings transferred to darkness for 0, 2 and 4 DDI. GAPDH was used as a control. DDI indicates day(s) of dark incubation. Data are means±s.d. of four biological replicates. * P <0.05, ** P <0.01 (Student’s t -test). Full size image To further explore how PIF4/PIF5 regulate the expression of SAGs, we tested whether the 132 shared DEGs include direct targets of PIF4/PIF5 transcription factors. Thirty two of the shared DEGs are PIF-direct targets ( P =0.0062, hypergeometric test), according to previously reported PIF4/PIF5 chromatin immunoprecipitation (ChIP)-seq data [34] , [40] . Their promoters are enriched with the G-box element (CACGTG), a typical binding motif for PIF transcription factors [34] , [40] , [41] , [42] , [43] ( Fig. 4b , upper panel). In contrast, the promoters of the indirectly regulated DEGs are enriched with ABRE-like elements (YACGT), the known binding sites of bZIP transcription factors, such as the positive ABA signalling component ABI5 [44] ( Fig. 4b , lower panel). These results suggest that PIF4/PIF5 directly activate the expression of many SAGs and also indirectly function through ABA signalling. Ethylene signalling also promotes senescence [13] , [14] , [15] , [16] ; we thus examined whether PIF4/PIF5 activate both ABA and ethylene signalling for inducing senescence. The GSEA indicated that both ABA- and ethylene-induced genes are downregulated in pifQ mutants at 2 DDI and are upregulated in senescing WT ( Supplementary Table 1 ). The suppression of ABA and ethylene signalling in pifQ mutants might be partly due to the decreased expression of EIN3 (a positive ethylene signalling component) and the Group A bZIP transcription factors ABI5 and EEL ( Fig. 4c,d,h–j ), which are direct targets of PIF4/PIF5, as shown by ChIP assays ( Fig. 4d ). Consistent with the decreased expression of ABI5 , EEL and EIN3 in pifQ mutants, the bZIP- and EIN3-induced genes, which were identified from previously reported microarray data (see Methods), were significantly downregulated in pifQ mutants and upregulated in senescing WT ( Supplementary Table 1 ). We found that abi5, eel and ein3 mutations delayed senescence, and abi5 and eel mutations showed additive effects ( Fig. 4e–g ), further supporting the hypothesis that decreased expression of ABI5 , EEL and EIN3 is closely associated with delayed senescence in pifQ mutants. Since ELF3 delays senescence by repressing the transcription of PIF4/PIF5 ( Fig. 3f ), ELF3 should repress the expression of ABI5 , EEL and EIN3 during dark incubation. Indeed, their mRNA expression was severely downregulated in ELF3 -OX plants and upregulated in elf3 mutants ( Fig. 4h–j ). These results indicate that PIF4/PIF5 regulate senescence partly through the two bZIPs and EIN3. PIF4/PIF5 activate ORE1 through multiple feed-forward loops We next investigated if PIF4, PIF5 and their direct target transcription factors (ABI5, EEL and EIN3) jointly affect the expression of known senescence-promoting regulators. To date, 3,744 senescence-associated loci in Arabidopsis have been curated [3] , and 89 loci are known to promote senescence. Among the 89 senescence-promoting genes [3] ( Supplementary Data 1 ), we found that ORE1 , encoding a key senescence-promoting NAC transcription factor, was commonly induced by all three groups of transcription factors ( Fig. 5a ). ORE1 expression was downregulated in ELF3 -OX plants and pifQ , abi5 , eel and ein3 mutants, and upregulated in elf3 mutants and PIF4 -OX plants ( Fig. 5b ), indicating that ORE1 is a target senTF acting downstream of ELF3 , PIF4, PIF5 , ABI5 , EEL and EIN3 . Consistent with this, ore1 mutants, similar to phyB and pif4 mutants, did not respond to red light pulse treatment during dark incubation ( Fig. 5c,d ). These results indicate that ORE1 integrates phyB-mediated light signalling to promote senescence in light-deprived conditions. 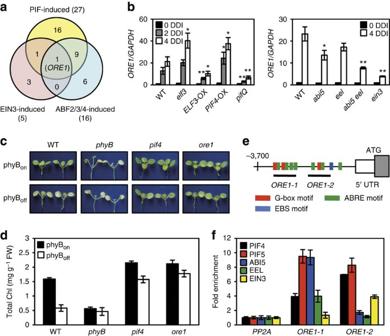Figure 5: PIF4/PIF5 induceORE1through multiple feed-forward loops. (a) Identification ofORE1as a common target of PIFs, bZIPs and EIN3. Among the literature-curated senescence-promoting genes3, DEGs (FDR<0.05) were identified from the microarray data for PIF-induced genes (this study), ABF2/3/4-induced genes67and EIN3-induced genes (GSE21762). (b) Regulation ofORE1expression by ELF3, PIF4/PIF5, ABI5, EEL and EIN3.ORE1mRNA levels were determined by quantitative real-time PCR at 0 (black bars), 2 (grey bars) and 4 (white bars) DDIs. GAPDHwas used as a control. Data are means±s.d. of at least four independent biological replicates. (c,d) Senescence induction in phyBoffconditions requiresORE1. Light-grown 7-day-old seedlings were transferred to darkness for 16 days with intermittent red light pulses (phyBon) or red/far-red light pulses (phyBoff) as shown inFig. 1aand total Chl levels (d) were measured to determine the degree of senescence. Data are means±s.d. of four biological replicates. (e) A diagram of theORE1promoter showing the positions of G-box elements (red boxes), ABRE-like elements (green boxes), EIN3 binding sites (EBS; blue box) and two ChIP amplicons (ORE1-1andORE1-2; black horizontal lines). (f) Direct binding of PIF4, PIF5, ABI5, EEL and EIN3 to theORE1promoterin vivo. Enrichment ofORE1promoter by PIF4 (black), PIF5 (red), ABI5 (blue), EEL (green) and EIN3 (yellow) were examined by ChIP-qPCR. Values were normalized to the values forPP2A, a non-binding control. Data are means±s.d. of two biological replicates. *P<0.05, **P<0.01 (Student’st-test). Figure 5: PIF4/PIF5 induce ORE1 through multiple feed-forward loops. ( a ) Identification of ORE1 as a common target of PIFs, bZIPs and EIN3. Among the literature-curated senescence-promoting genes [3] , DEGs (FDR<0.05) were identified from the microarray data for PIF-induced genes (this study), ABF2/3/4-induced genes [67] and EIN3-induced genes (GSE21762). ( b ) Regulation of ORE1 expression by ELF3, PIF4/PIF5, ABI5, EEL and EIN3. ORE1 mRNA levels were determined by quantitative real-time PCR at 0 (black bars), 2 (grey bars) and 4 (white bars) DDIs . GAPDH was used as a control. Data are means±s.d. of at least four independent biological replicates. ( c , d ) Senescence induction in phyB off conditions requires ORE1 . Light-grown 7-day-old seedlings were transferred to darkness for 16 days with intermittent red light pulses (phyB on ) or red/far-red light pulses (phyB off ) as shown in Fig. 1a and total Chl levels ( d ) were measured to determine the degree of senescence. Data are means±s.d. of four biological replicates. ( e ) A diagram of the ORE1 promoter showing the positions of G-box elements (red boxes), ABRE-like elements (green boxes), EIN3 binding sites (EBS; blue box) and two ChIP amplicons ( ORE1-1 and ORE1-2 ; black horizontal lines). ( f ) Direct binding of PIF4, PIF5, ABI5, EEL and EIN3 to the ORE1 promoter in vivo . Enrichment of ORE1 promoter by PIF4 (black), PIF5 (red), ABI5 (blue), EEL (green) and EIN3 (yellow) were examined by ChIP-qPCR. Values were normalized to the values for PP2A , a non-binding control. Data are means±s.d. of two biological replicates. * P <0.05, ** P <0.01 (Student’s t -test). Full size image We found that the ORE1 promoter harbours three potential PIF binding sites (G-box motifs), several bZIP binding sites (ABRE motifs) and an EIN3 binding site ( Fig. 5e ), suggesting that ORE1 is a direct target of not only PIF4/PIF5 but also of bZIPs and EIN3. To examine whether PIF4, PIF5, ABI5, EEL and EIN3 directly activate ORE1 transcription, we next performed ChIP assays and found that all of the tested TFs bind to the ORE1 promoter ( Fig. 5f ). Collectively, the direct activation of ORE1 transcription by PIF4/PIF5 and by PIF4/PIF5-targeted transcription factors (ABI5, EEL and EIN3) indicates that these transcription factors establish multiple coherent feed-forward regulatory loops to induce leaf senescence; PIF4/PIF5 directly activate the expression of ABI5, EEL and EIN3 , and in turn, PIF4, PIF5, ABI5, EEL and EIN3 directly activate ORE1 transcription. ABI5 and EEL directly promote Chl degradation PIF4, PIF5 and their direct target transcription factors (EIN3 and bZIPs) may have other senescence-related targets in addition to ORE1 . Microarray data analysis indicated that among the SAGs, PIF4, PIF5 and bZIPs induce four Chl catabolism-associated genes, including STAYGREEN 1 ( SGR1 , also known as NYE1 ) and NON-YELLOW COLORING 1 ( NYC1 ) (refs 45 , 46 ) ( Supplementary Table 2 ). SGR1 and NYC1 expression was downregulated in ELF3 -OX plants and pifQ mutants, and upregulated in elf3 mutants and PIF4 -OX plants ( Fig. 6a ). We also found the bZIP binding motif (ABRE motif) in the promoters of SGR1 and NYC1 ( Fig. 6b ). Consistent with the presence of ABREs, ChIP assays revealed that ABI5 and EEL directly bind to the promoters of SGR1 and NYC1 ( Fig. 6c ) and the expression levels of SGR1 and NYC1 were significantly downregulated in abi5 eel double mutants during DIS ( Fig. 6d ). Although the promoters of SGR1 and NYC1 also contain a putative PIF binding motif (G-box motif; Supplementary Fig. 11a ), PIF4/PIF5 did not bind to the G-box motifs of SGR1 and NYC1 ( Supplementary Fig. 11b ). The results indicate that PIF4/PIF5 indirectly promote Chl degradation through their target bZIPs during leaf senescence. 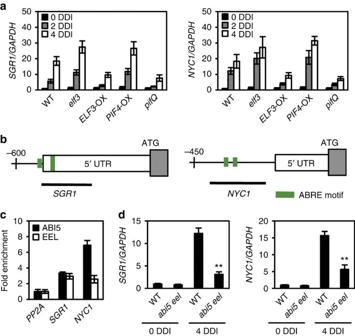Figure 6: bZIPs directly induceSGR1andNYC1for Chl breakdown. (a) Gene expression analysis ofSGR1andNYC1in light-grown 7-day-old WT (Col),elf3(elf3-8),ELF3-OX,pifQandPIF4-OX plants at 0, 2 and 4 DDI. (b) The promoter regions ofSGR1andNYC1showing the position of ABRE motifs (green boxes) and ChIP amplicons (black thick underlines). (c) ChIP assays showing direct binding of ABI5 and EEL to the promoters ofSGR1andNYC1. ThePP2Alocus was used as a non-binding control. Data are means±s.d. of two independent biological replicates. (d) Decreased expression ofSGR1andNYC1inabi5 eeldouble mutants. Gene expression was measured by quantitative real-time PCR using light-grown 7-day-old seedlings transferred to darkness for 0 and 4 days. The relative mRNA levels ofSGR1andNYC1were normalized toGAPDHexpression as a control. Data are means±s.d. of four independent biological replicates. **P<0.01 (Student’st-test). Figure 6: bZIPs directly induce SGR1 and NYC1 for Chl breakdown. ( a ) Gene expression analysis of SGR1 and NYC1 in light-grown 7-day-old WT (Col), elf3 ( elf3-8 ), ELF3 -OX, pifQ and PIF4 -OX plants at 0, 2 and 4 DDI. ( b ) The promoter regions of SGR1 and NYC1 showing the position of ABRE motifs (green boxes) and ChIP amplicons (black thick underlines). ( c ) ChIP assays showing direct binding of ABI5 and EEL to the promoters of SGR1 and NYC1 . The PP2A locus was used as a non-binding control. Data are means±s.d. of two independent biological replicates. ( d ) Decreased expression of SGR1 and NYC1 in abi5 eel double mutants. Gene expression was measured by quantitative real-time PCR using light-grown 7-day-old seedlings transferred to darkness for 0 and 4 days. The relative mRNA levels of SGR1 and NYC1 were normalized to GAPDH expression as a control. Data are means±s.d. of four independent biological replicates. ** P <0.01 (Student’s t -test). Full size image Light deprivation initiates leaf senescence in plants. In this study, we reveal the molecular genetic pathway by which light deprivation accelerates senescence, via increased levels of PIF4/PIF5 mRNAs and PIF4/PIF5 proteins, which are negatively regulated by ELF3 and phyB, respectively ( Fig. 7 ). The increased activity of PIF4/PIF5 promotes the expression of ORE1 not only by directly binding to its promoter but also indirectly through EIN3 and bZIPs (ABI5 and EEL). These TFs, in turn, activate the expression of hundreds of SAGs that mediate the highly ordered decomposition of cellular components, such as Chls and photosynthetic proteins in chloroplasts, finally leading to leaf senescence [1] , [3] , [4] . 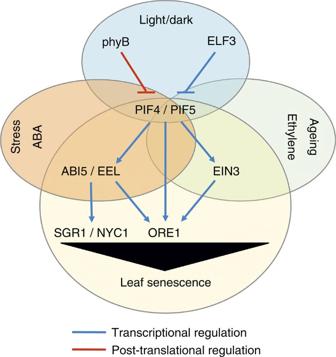Figure 7: A proposed model for PIF4/PIF5-induced leaf senescence. PIF4/PIF5 promote DIS by forming multiple coherent feed-forward loops with bZIPs (ABI5andEEL),EIN3andORE1, all of which are inhibited by phyB and ELF3. Figure 7: A proposed model for PIF4/PIF5-induced leaf senescence. PIF4/PIF5 promote DIS by forming multiple coherent feed-forward loops with bZIPs ( ABI5 and EEL ), EIN3 and ORE1 , all of which are inhibited by phyB and ELF3. Full size image We used plate-grown young seedlings rather than adult plants for the majority of the senescence assays, because it is easier to synchronize the growth of seedlings and to reduce unknown variation caused by environmental fluctuations. However, as we have shown, phyB and elf3 mutants senesce early, while pif4 , pif5 and pifQ mutants senesce later, not only in seedlings but also in detached, attached or individually covered leaves of adult plants, suggesting that the senescence pathways identified in seedlings are likely important for senescence at other stages of development. Overall, our data show that PIF4/PIF5 promote senescence throughout development, while phyB and ELF3 repress PIF4/PIF5 to prevent precocious senescence in the presence of light. Our study revealed the role of PIF4/PIF5 in senescence in relation to light signalling, and other works showed that PIF4 also mediates high temperature signalling to promote hypocotyl growth [47] . Thus, additional work is required to investigate whether other signals from abiotic stresses, such as high temperature, also regulate senescence through PIF4/PIF5. The identified pathway links light signalling to senescence and consists of multiple coherent feed-forward loops, which likely function to make the pathway robust. In conditions with sufficient light, ELF3 and phyB convey light information to PIF4/PIF5, resulting in the reduction of PIF4/PIF5 mRNA and protein levels ( Figs 2g and 3f ). Under prolonged darkness, however, the process reverses and PIF4/PIF5 mRNA and protein levels increase. The increased PIF4/PIF5 activate the expression of EIN3 and two bZIPs ( ABI5 and EEL ) by directly associating with their promoters ( Fig. 4c,d,h–j ), thus affecting regulators of ethylene and ABA signalling, respectively. In turn, the increased EIN3 and bZIPs directly activate the expression of ORE1 ( Fig. 5f ), a major senescence-promoting NAC transcription factor that regulates hundreds of SAGs. Notably, not only EIN3 and bZIPs but also PIF4/PIF5 directly bind to the ORE1 promoter to activate its expression ( Fig. 5f ), indicating that PIF4/PIF5 form coherent feed-forward loops to activate the expression of ORE1 ( Fig. 7 ). Such coherent feed-forward loops make a pathway less prone to being disturbed by ephemeral environmental fluctuations [48] . Similar coherent feed-forward loops between EIN2 and ORE1 were previously proposed [5] ; EIN2 activates the expression of ORE1 both by repressing the expression of miR164 , which cleaves the ORE1 mRNA, and by a miR164 -independent pathway. EIN2 also inhibits the expression of miR164 through EIN3, which directly binds to the miR164 promoter [17] . Since we showed that EIN3 directly binds to the ORE1 promoter to activate its expression ( Fig. 5b,f ), these results suggest that a previously proposed miR164 -independent pathway likely functions through EIN3 and thus EIN3 , miR164 , and ORE1 form a coherent feed-forward loop. Such a loop implies that the cascade of coherent feed-forward loops regulates the expression of ORE1 during senescence. We note that EIN3 also directly binds to the promoter of NAP , a major senescence-promoting NAC transcription factor and one of the 89 senescence-promoting genes [3] ( Supplementary Data 1 ), and induces NAP transcription [49] , indicating that EIN3 activates the expression of both ORE1 and NAP . Our study showed that ELF3 represses senescence independently of its previously reported roles in light signalling. A previous study showed that ELF3 interacts with phyB to regulate the phyB signal transduction pathway [35] . Although ELF3 represses senescence as phyB does, the elf3 mutants still respond to red light pulse treatment similar to WT, indicating that ELF3 regulates senescence independent of phyB activity [35] , [50] . The fact that ELF3 represses the expression of PIF4/PIF5 mRNA and phyB promotes the degradation of PIF4/PIF5 proteins further supports the independent roles of ELF3 and phyB in senescence ( Figs 2g and 3f ). Our study also suggests that ELF3 represses senescence independently of its roles in circadian clock, flowering time and diurnal control of hypocotyl elongation. First, ELF3 is required to maintain the circadian clock under continuous light [51] and its mRNA expression is directly repressed by CCA1 for the regulation of the diurnal control of hypocotyl length and flowering time [52] . Besides elf3 mutants, however, the circadian-clock mutants including cca1 , lhy1 and det1 do not exhibit an altered senescence phenotype in darkness ( Supplementary Fig. 8b ), indicating that the dysfunction of the circadian clock per se does not cause the early senescence symptoms of elf3 mutants. Second, ELF3 interacts with COP1, which allows COP1 to destabilize GI downstream of CRY2 to control flowering time [36] . However, cop1 , gi , fkf1 , co and cry2 mutants do not show any senescence-associated phenotype in darkness, suggesting that the flowering-time defect in elf3 mutants is irrelevant to the early senescence in darkness. Third, ELF3 forms an evening complex with ELF4 and LUX and represses the expression of PIF4/PIF5 mRNAs for diurnal control of hypocotyl elongation [30] . Unlike the elf3 mutants, elf4 and lux mutants senesce at the same rate as WT in darkness, indicating that ELF3 acts as the transcription repressor of PIF4/PIF5 in the absence of ELF4 or LUX. Taken together, our data suggest that the inhibition of senescence represents a novel function of ELF3. The increase of PIF4/PIF5 expression independent of phyB ( Fig. 2f ) raises the possibility that other light signalling components also suppress senescence by repressing the expression of PIF4/PIF5 in connection with ELF3. A previous study showed that ELF3 is destabilized when light-grown seedlings were transferred to darkness [35] . It is not known, however, which light signalling components regulate ELF3 stability. A few possibilities exist. First, the inactivation of other phytochromes might be responsible for the destabilization of ELF3, which leads to the upregulation of PIF4/PIF5 expression in the dark, but the role of phyA in senescence remains inconclusive. We showed that the Arabidopsis phyA mutants do not show any senescence phenotype in our conditions ( Supplementary Fig. 2 ). Unlike our analysis, however, other studies have reported two contradictory roles of phyA in senescence: the overexpression of oat phyA delayed senescence in tobacco [53] , whereas the pea phyA mutants exhibited delayed senescence [54] . These contrasting results could be due to the different senescence conditions (dark-induced versus natural senescence) or different plant species ( Arabidopsis versus tobacco versus pea). Alternatively, phyA proteins from different plant species might have different functions. For example, Arabidopsis phyA does not mediate the red light-low fluence response (LFR) [55] , whereas monocot phyA mediates the red light-LFR even when it is expressed in Arabidopsis [56] . Thus, the suppression of senescence by oat phyA could be due to its unique ability to mediate the LFR, a function usually reserved for phyB [57] . The delayed, rather than early, senescence of pea phyA mutants also excludes pea phyA as the repressor of PIF4/PIF5 mRNA expression in the dark. Currently, the role of three minor phytochromes (phyC, phyD and phyE) in senescence remains to be examined. Second, the activation of the expression of PIF4/PIF5 during senescence might require the absence of blue light, rather than presence of red light. Previous studies showed that blue light pulses inhibit DIS in papaya [58] . In soybean, CRY2a interacts with and inhibits a CRY-interacting CRYPTOCHROME-INTERACTING BASIC-HELIX-LOOP-HELIX 1 (CIB1) transcription factor that promotes leaf senescence by directly upregulating the expression of WRKY53 (ref. 59 ). Since low red to far-red ratio also promotes leaf senescence in soybean [60] , both phytochrome and cryptochrome signals can delay leaf senescence in soybean. However, we found that cryptochrome signalling does not regulate senescence in Arabidopsis ( Supplementary Fig. 8c ). Since blue light is perceived not only by CRY but also by phototropins and Light–Oxygen–Voltage-sensing-domain containing F-box proteins [23] , our data do not exclude the possibility that other blue light receptors repress senescence through ELF3. Further investigation is needed to determine which light signals regulate the expression of PIF4/PIF5 mRNA through ELF3 during senescence. The inclusion of ABI5 and EIN3 in the PIF4/PIF5-initiated feed-forward loops suggests that the identified regulatory loops integrate signals from light, abiotic stress and ageing, to regulate senescence ( Fig. 7 ). Previous studies showed that ABA signalling increases the activity of ABI5 and its homologues, Group A bZIPs, in response to abiotic stresses, both at the transcriptional and post-transcriptional levels [44] , [61] (AtGenExpress; abiotic stress). Activated ABI5 and its homologues trigger a subset of ABA responses, including senescence ( Fig. 4e–g ), seedling growth arrest and abiotic stress tolerance [61] , [62] . Our data indicate that PIF4/PIF5 also activate the expression of ABI5 and its homologues at the transcriptional level, by directly binding to their promoters ( Fig. 4c,d,h–j ). Light decreases the activity of PIF4/PIF5; this finding indicates that light and abiotic stresses antagonistically regulate the expression of ABI5 and its homologues. This finding also indicates that the integration of light and abiotic stress signalling determines the output of the PIF4/PIF5-initiated coherent feed-forward loops. Similarly, the PIF4/PIF5-initiated coherent feed-forward loops likely integrate developmental stage signals through EIN3, as shown by a gradual increase of EIN3 expression during ageing, and the consequent promotion of age-dependent senescence [16] . In conclusion, identification of EIN3 and ABI5 as constituents of the loops in our model suggests that light signalling (represented by PIF4/PIF5) interacts with abiotic stress signalling (ABI5 and EEL) [62] and developmental age signalling (EIN3) [16] to regulate senescence ( Fig. 7 ). The interplay among these signals provides the mechanism by which plants decide when to senesce in response to ageing and dynamic environmental conditions. Plant materials and growth conditions Arabidopsis thaliana plants were grown at 22 to 24 °C under long days (16-h light/8-h dark) in a growth room equipped with cool-white fluorescent light (90 to 100 μmol m −2 s −1 ) for general growth and seed harvest. For phenotypic analysis, surface-sterilized seeds were plated on Murashige and Skoog (MS) agar plates (half-strength MS, 0.8% phytoagar and 0.05% MES, pH 5.7) and stratified for 3 days at 4 °C in darkness before being transferred to the growth room. For DIS, 7-day-old seedlings, detached (4th or 5th) rosette leaves of 3-week-old plants with 3 mM MES buffer (pH 5.8) or whole plants were incubated in complete darkness for the indicated periods. For quantitative reverse transcriptase PCR and dark treatment with or without light pulse irradiance, 7-day-old seedlings grown on MS agar plates grown under continuous light (100 μmol m −2 s −1 ) were incubated in darkness with or without 5 min of red light (13 μmol m −2 s −1 ) followed by darkness or 5 min of far-red light (3.2 μmol m −2 s −1 ) for the indicated periods. Plasmid construction and plant transformation For Arabidopsis transgenic plants expressing genes under the control of the 35S promoter, the full-length PHYB , PIF4 , PIF5 , ABI5 , EEL and EIN3 cDNAs were amplified with specific primers ( Supplementary Table 4 ), cloned into the binary vectors, pBI121 ( PIF4 and PIF5 ) and pCAMBIA1300, bearing either GFP ( PHYB ), Myc ( PIF4 and PIF5 ) or FLAG ( ABI5 , EEL and EIN3 ) tag, and transformed into WT (Col-0) by Agrobacterium -mediated transformation. 35S:FLAG - ABI5 and 35S:FLAG-EEL are hypersensitive to ABA and 35S:EIN3-FLAG is hypersensitive to ethylene ( Supplementary Fig. 12 ). Measurement of Chl pigments For measurement of total Chl concentration, Chl pigments were extracted with 80% ice-cold acetone from leaf tissues of plants grown under long days. The Chl concentration was determined using an ultraviolet/visible spectrophotometer according to the previous method [63] . Reverse transcription and quantitative real-time PCR Total RNA from plant tissues was isolated using the Total RNA Extraction Kit (iNtRON Biotechnology, Korea). For RT, first-strand cDNAs were prepared with 5 μg of total RNA using M-MLV reverse transcriptase and oligo(dT) 15 primer (Promega) and diluted to 100 μl with water. Gene expression levels were determined by qPCR analysis. Twenty microlitres of qPCR mixture contained 2 μl of first-strand cDNAs, 10 μl of 2X QuantiTect SYBR Green I Master (Roche) and 0.25 μM of the forward and reverse primers for each gene. The qPCR analysis was performed using the Light Cycler 2.0 (Roche Diagnostics). Relative expression levels of each gene were normalized to mRNA levels of glyceraldehyde phosphate dehydrogenase ( GADPH ) as a loading control. The gene-specific primers for qPCR are listed in Supplementary Table 4 . Measurement of ion leakage rate To measure ion leakage rate caused by DIS, approximately 10 whole seedlings or 10 rosette leaves in each condition were placed in a tube with 6 ml of 0.4 M mannitol solution. The tubes were placed at room temperature for 3 h with gentle shaking. Conductivity of incubated solution was measured before and after boiling for 10 min, using an electroconductivity metre (CON6 METRE, LaMOTTE Co., USA). The ion leakage rate was calculated by the ratio of initial to total conductivity. SDS-PAGE and immunoblot analysis PIF4-Myc and PIF5-Myc seedlings were collected and immediately frozen in liquid nitrogen under a dim green light. The seedlings were then ground in liquid nitrogen and homogenized in denaturing buffer (100 mM NaH 2 PO 4 , 10 mM Tris-HCl, 8 M urea, pH 8.0) by vigorous vortexing. The debris was removed by centrifugation at 20,000 g for 10 min at 4 °C. For immunoblot analysis, the supernatants were separated on an 8% SDS-polyacrylamide gel, and the proteins were transferred to a nitrocellulose membrane (Hybond ECL, Amersham) using transfer buffer (5.8 g l −1 Tris base, 29 g l −1 glycine, 20% methanol and 0.01% SDS). For protein detection, rabbit polyclonal anti-Myc antibody (Santa Cruz, USA) with 1/1,000 dilution for PIF4-Myc and PIF5-Myc and mouse monoclonal anti-tubulin antibody (Sigma, USA) with 1/10,000 dilution for a loading control in PBS buffer containing 0.05% Tween 20 were used. Blots were washed three times with the same buffer and then incubated with appropriate secondary antibodies. After washing three times, the horseradish peroxidase activity of secondary antibodies was detected using an ECL detection kit (AbFRONTIER, Korea). Uncropped blot images of Fig. 2g are shown in Supplementary Fig. 13 . Microarray analysis For microarray analysis, 7-day-old light-grown seedlings of WT and pifQ mutants were incubated in the dark for 2 days before RNA extraction. Total RNA was extracted using the Spectrum Plant Total RNA kit (Sigma-Aldrich, USA). Three biological replicates of WT and pifQ mutants were grown and sampled for RNA purification. Two μg of total RNA was used for probe synthesis. The Agilent Arabidopsis Genome 44 K chip (version 4) was used. The analysis of microarray data was done in R version 2.15.0. The limma package was used for background correction and for normalization within arrays and between arrays [64] . Then, a linear model was fitted using lmFit followed by statistical calculation using ebayes . FDR less than 0.05 was applied to identify DEGs. Microarray data were deposited in the NCBI Gene Expression Omnibus (GEO) with accession number GSE52646 . For the identification of DEGs of WT DIS and hormonal transcription factor-activated genes, raw data deposited in NCBI GEO and EMBL-EBI were obtained and processed as described above. ChIP assay The plants overexpressing PIF4-Myc , PIF5-Myc , ABI5-FLAG , EEL-FLAG and EIN3-FLAG under the cauliflower mosaic virus 35S promoter (see Plasmid construction and plant transformation) were grown in continuous white light for 7 days and then transferred to darkness for 3 days before cross-linking for 20 min with 1% formaldehyde under vacuum. Chromatin complexes were isolated and sonicated with slight modification [43] . Anti-Myc monoclonal antibody (mouse, Cell Signaling) or anti-FLAG polyclonal antibody (rabbit, Sigma), and Protein A agarose/salmon sperm DNA (Millipore) were used for immunoprecipitation. After reverse cross-linking and protein digestion, DNA was purified by QIAquick PCR Purification Kit (Qiagen). GSEA GSEA [65] was conducted with Software GSEA v2.08 (Broad Institute, MIT) according to the online user guide ( http://www.broadinstitute.org/gsea ). ABA and ACC-responsive gene sets were generated based on previously processed microarray data [66] . Sets of genes activated by ABI5, ABF2/3/4 and EIN3 were identified from public microarray data from previous studies [67] , [68] and from NCBI GEO deposition (GSE21762) with twofold criteria (FDR<0.05) as described in Microarray Analysis. The set of genes activated by ABI5 was further selected for genes whose expression is induced by ABA treatment (AtGenExpress). Parameters were set as gene_set for permutation type, 1,500 for maximal size of gene set and default for other parameters. Y.S., J.J., M.-Y.K. and J.K. performed the experiments. N-C.P. and G.C. designed the study and supervised the work. All authors discussed the results and made substantial contributions to the manuscript. How to cite this article: Sakuraba, Y. et al . Phytochrome-interacting transcription factors PIF4 and PIF5 induce leaf senescence in Arabidopsis . Nat. Commun. 5:4636 doi: 10.1038/ncomms5636 (2014). Accession codes: Gene information from this article can be found in the Arabidopsis Genome Initiative or GenBank/EMBL databases as the following accession numbers: ABI5 , At1g16540 ; CO , At5g15840 ; CRY1 , At4g08920 ; CRY2 , At1g04400 ; DET1 ; At4g10180 ; EEL , At1g30230 ; EIN3 , At3g20770 ; ELF3 , At2g25930 ; ELF4 , At2g40080 ; GAPDH , At3g26650 ; Lhcb1 , At1g29910 ; LUX , At3g46640 ; NYC1 , At4g13250 ; ORE1 , At5g39610 ; PHYA , At1g09570 ; PHYB , At2g18790 ; PIF1 , At2g20180 ; PIF3 , At1g09530 ; PIF4 , At2g43010 ; PIF5 , At3g59060 ; PIL1 , At2g46970 ; PP2A , At1g13320 ; RGA , At2g01570 ; SAG12 , At5g45890 ; SEN4 , At4g30270 ; SGR1 , At4g22920 . Microarray data were deposited in the NCBI Gene Expression Omnibus (GEO) with accession number GSE52646 .